Genome engineering empowers the diatomPhaeodactylum tricornutumfor biotechnology Diatoms, a major group of photosynthetic microalgae, have a high biotechnological potential that has not been fully exploited because of the paucity of available genetic tools. Here we demonstrate targeted and stable modifications of the genome of the marine diatom Phaeodactylum tricornutum , using both meganucleases and TALE nucleases. When nuclease-encoding constructs are co-transformed with a selectable marker, high frequencies of genome modifications are readily attained with 56 and 27% of the colonies exhibiting targeted mutagenesis or targeted gene insertion, respectively. The generation of an enhanced lipid-producing strain (45-fold increase in triacylglycerol accumulation) through the disruption of the UDP-glucose pyrophosphorylase gene exemplifies the power of genome engineering to harness diatoms for biofuel production. Diatoms, a phylogenetic group comprising 10,000 to 100,000 different species, are unicellular photoautotrophic algae that play a major role in the global ecosystem by fixing atmospheric CO 2 in the oceans [1] . Through photosynthesis, diatoms produce more than 20% of the oxygen generated on earth, a contribution equivalent to that of all the world’s rainforests [2] , [3] . They also participate in the biogeochemical cycling of dissolved silicates by integrating them into their highly structured cell walls called frustules [4] . Besides the substantial role diatoms play in the maintenance of the global ecosystem, they also offer huge biotechnological advantages [5] , [6] . Their highly structured mesoporous cell wall of amorphous silica can be incorporated directly into nanodevices or used for the bioencapsidation and delivery of molecules [7] . Furthermore, diatoms are coveted organisms in the pharmaceutical, cosmetic and food industries as a natural source of polyunsaturated fatty acids, pigments and antioxidants [8] , [9] , [10] , [11] . Diatoms can also be used as expression systems for recombinant proteins or biomaterials [12] , [13] . However, due to the increasing scarcity of fossil fuels, their major potential probably lies in the production of biofuels [14] . The wide diversity of fatty acids produced by diatoms, and their capacity to accumulate lipids during dormancy or after stress, makes them organisms of choice for biofuel production [15] , [16] , [17] . Trentacoste et al. [18] have recently shown the potential of the diatom Thalassiosira pseudonana for biofuel production using RNA interference (RNAi) and antisense approaches. Although the genomes of several diatom species have been sequenced and publicly released [19] , the use of these species as industrial biofactories has been hampered by the paucity of genome engineering tools. The diploid genome and unknown sexual lifecycle of model species has impeded classical approaches to genetic improvement based on random mutagenesis and phenotypic selection. Furthermore, the generation of strains with modulated gene expression relies mainly on random integration of transgenes to achieve overexpression or targeted gene silencing using RNAi [20] , [21] . One improvement would be targeted gene insertion (TGI) for overexpression via homologous recombination (HR), as demonstrated in Nannochloropsis [22] and Chlamydomonas reinhardtii using zinc-finger nuclease technology [23] . However, to our knowledge, genome modification by HR has never been reported in diatoms. Zinc-finger nucleases, meganucleases (MNs), transcription activator-like effector nucleases (TALEN) and clustered regularly interspaced short palindromic repeats (CRISPR/Cas9) have emerged during the past decade as efficient tools for genome editing in many organisms [24] , [25] . These molecular scissors are able to introduce a targeted DNA double-strand break that is repaired by one of two major mechanisms: non-homologous end-joining, which leads to gene disruption by inducing mutations at the break site, or homologous recombination, which drives gene insertion or gene replacement using exogenous DNA templates with homology to the targeted locus ( Fig. 1a ). The use of sequence-specific nucleases has been reported to stimulate up to 1,000-fold the HR frequency [26] , which prompted us to investigate their potential for diatom genome engineering. 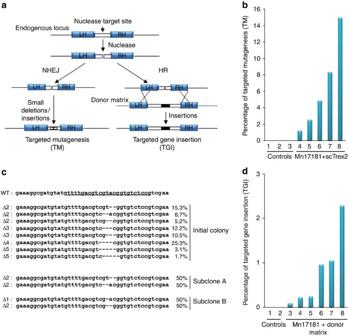Figure 1: Genotypic characterization of strains engineered using nucleases. (a) Overview ofin vivodouble-strand break repair mechanisms by non-homologous-end-joining (NHEJ) and homologous recombination (HR), resulting in disruption of the nuclease target site either by targeted mutagenesis (*) or targeted gene insertion (black rectangle). For TGI, the donor matrix consisted of two homologous regions of 750 bp each (LH, left homology; RH, right homology) flanking a 29-bp insertion. (b) Targeted mutagenesis (TM) frequencies induced by the meganuclease Mn17181 in combination with the DNA-processing enzyme scTrex2 (colonies 4 to 8). Events were quantified via amplicon sequencing using primers surrounding the nuclease target site. All the transformants were obtained by co-transformation with the plasmid conferring resistance to the nourseothricin antibiotic. The baseline controls correspond to clones transformed with a plasmid carrying the antibiotic resistance gene alone (colonies 1 to 3). (c) Nature of mutagenic events induced by Mn17181 in the mosaic colony and its derivative subclones. The sequence underlined corresponds to the recognition site of Mn17181. In the top panel are the main mutagenic events present in the colony harbouring 15% TM. The percentage of each event is indicated on the right. On the left, the size of deletion is indicated after the symbol (Δ). In the bottom panel are two subclones (A and B) harbouring targeted mutations on both alleles. In the case of subclone B, sequencing revealed the 1-bp deletion, which was discarded by filtering deep sequencing reads as presented inSupplementary Fig. 6. (d) Targeted gene insertion (TGI) frequencies induced by meganuclease Mn17181 in the presence of the donor matrix (colonies 3–8) as measured by deep sequencing. The baseline controls correspond to colonies transformed with a plasmid carrying the antibiotic resistance gene in the presence of the donor matrix (colonies 1 and 2). TGI frequencies induced by Mn17181 were measured by deep sequencing. Figure 1: Genotypic characterization of strains engineered using nucleases. ( a ) Overview of in vivo double-strand break repair mechanisms by non-homologous-end-joining (NHEJ) and homologous recombination (HR), resulting in disruption of the nuclease target site either by targeted mutagenesis (*) or targeted gene insertion (black rectangle). For TGI, the donor matrix consisted of two homologous regions of 750 bp each (LH, left homology; RH, right homology) flanking a 29-bp insertion. ( b ) Targeted mutagenesis (TM) frequencies induced by the meganuclease Mn17181 in combination with the DNA-processing enzyme scTrex2 (colonies 4 to 8). Events were quantified via amplicon sequencing using primers surrounding the nuclease target site. All the transformants were obtained by co-transformation with the plasmid conferring resistance to the nourseothricin antibiotic. The baseline controls correspond to clones transformed with a plasmid carrying the antibiotic resistance gene alone (colonies 1 to 3). ( c ) Nature of mutagenic events induced by Mn17181 in the mosaic colony and its derivative subclones. The sequence underlined corresponds to the recognition site of Mn17181. In the top panel are the main mutagenic events present in the colony harbouring 15% TM. The percentage of each event is indicated on the right. On the left, the size of deletion is indicated after the symbol (Δ). In the bottom panel are two subclones (A and B) harbouring targeted mutations on both alleles. In the case of subclone B, sequencing revealed the 1-bp deletion, which was discarded by filtering deep sequencing reads as presented in Supplementary Fig. 6 . ( d ) Targeted gene insertion (TGI) frequencies induced by meganuclease Mn17181 in the presence of the donor matrix (colonies 3–8) as measured by deep sequencing. The baseline controls correspond to colonies transformed with a plasmid carrying the antibiotic resistance gene in the presence of the donor matrix (colonies 1 and 2). TGI frequencies induced by Mn17181 were measured by deep sequencing. Full size image Here we report high frequencies of targeted genome modification in diatoms using two types of designer nucleases, MNs and TALE nucleases. We use these nucleases to induce targeted mutagenesis (TM) of several genes involved in lipid metabolism, allowing us to generate a diatom strain exhibiting a 45-fold increase in triacylglycerol accumulation, while simultaneously reducing production costs. Targeted genome modifications induced by MNs We began with I-CreI-derived MNs delivered as monomeric proteins, which often make MN-encoding constructs easier to introduce into cells. Given the low transformation efficiency achieved in diatoms by the particle bombardment method used in most laboratories, we hypothesized that MNs were the best candidate to initiate our genome engineering efforts. An examination of the recently published genome sequence of Phaeodactylum tricornutum (Pt) enabled the identification of loci targetable by two existing engineered MNs (Mn17181 and Mn17038) from our proprietary collection. The ability of MNs to induce TM was assessed by co-transforming Pt with a MN-encoding plasmid, an autonomous selection cassette plasmid ( NAT gene to select for nourseothricin (NAT) resistance), and a plasmid encoding the DNA processing enzyme scTrex2, which has previously been shown to increase about 10-fold the TM frequency induced by MNs in mammalian cells [27] , [28] . Twelve NAT-resistant colonies transformed with Mn17181 were analysed for the presence of mutations using locus-specific PCR followed by deep sequencing. Of those colonies, 42% (5/12) exhibited TM and harboured both the plasmids encoding scTrex2 and meganuclease ( Supplementary Table 1 ). Every colony was mosaic, that is, composed of a mixture of cells with or without mutations. Depending on the colony, from 1 to 15% of the cells had targeted mutations ( Fig. 1b ). Mosaicism has been described by Seligman et al. [29] in the yeast Saccharomyces cerevisiae, where sectored colonies arose due to the cleavage activity of variants of the I-CreI-homing endonuclease. Indeed, mutagenesis does not necessarily occur within the initially transformed cell, but rather can occur during the subsequent cell divisions, as the majority of the double-strand breaks induced by the nucleases are repaired by faithful re-ligation without incorporating mutations. Therefore, each colony can be a mixed population of cells with or without mutations and with mutations of different types. We thus subcloned colonies to isolate and identify cells with bi-allelic mutations. We observed bi-allelic mutations in 29% (7/24) of the subclones derived from a colony with 15% overall TM. In agreement with our previous study on the processivity of the scTrex2 exonuclease [27] , small deletions of 1 to 4 nucleotides were predominantly found at the double-strand break site ( Fig. 1c ). We next asked whether Mn17181 could also drive efficient TGI via homologous recombination. For this purpose, the Pt strain was co-transformed with the Mn17181-encoding plasmid and a donor template carrying two homology arms with sequence identity to the targeted locus. 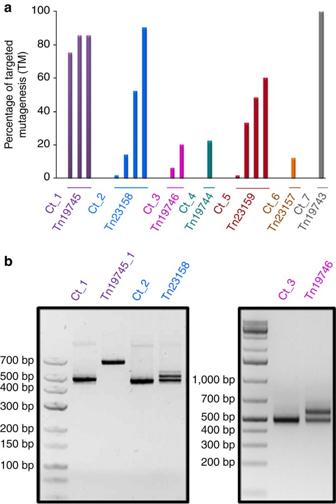Figure 2: Targeted mutagenesis induced by TALE nucleases. (a) TM frequency induced by TALEN-targeting genes involved in lipid metabolism and measured by deep sequencing. All the colonies with targeted mutations after transformation with their respective TALEN (Supplementary Table 4) are represented in this graph. Mutations were detected via amplicon sequencing using primers flanking the nuclease target site. For each locus, the control corresponds to a colony transformed with a plasmid carrying the antibiotic resistance gene alone (Ct_1 to Ct_7). (b) Examples of mutagenic events induced by TALEN Tn19745, Tn23158 and Tn19746, and directly evidenced by the presence of higher PCR products when compared with their respective controls (Ct_1 to Ct_3). A total of 22 NAT-resistant colonies were obtained, of which 27% (6/22) had TGIs ( Supplementary Table 2 ). Again, the colonies were heterogeneous, and the number of cells with TGI in a given colony ranged from 0.08 to 2.3% ( Fig. 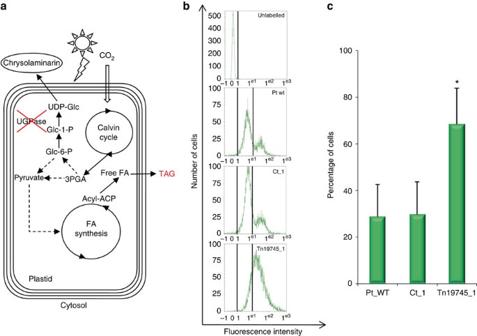Figure 3: Analysis of neutral lipid profiles by flow cytometry. (a) Simplified overview of the pathways involved in fatty acid synthesis and chrysolaminarin accumulation. (b) Flow cytometry analysis of neutral lipid content in the UGPase knock-out clone (Tn19745_1), a clone transformed with the plasmid for nourseothricin resistance (Ct_1) and the Pt parental strain (Pt wt). This BODIPY profile corresponds to one of the four experiments quantified inc. The graph represents the number of cells as a function of the fluorescence intensity of BODIPY labelling. Vertical lanes delimit, on the left, the fraction of the unlabelled cells, and, on the right, the fraction of cells exhibiting low versus high fluorescence intensity, which refers to cells with low versus high neutral lipid content. (c) Quantification of the number of cells with high-lipid content was performed in four independent experiments with Tn19745_1 compared with Pt wt (t-test, *P<0.05) and Ct_1 (t-test, *P<0.05). Data are shown as the mean+s.d. 1d and Supplementary Table 3 ). Genetically homogenous subclones could readily be obtained. The TGI results highlight that the machinery to carry out HR is preserved in diatoms, and this will allow for other genome modifications including gene replacements. No TGI were detected in the absence of the nuclease, demonstrating that a double-strand break was required for efficient HR in the Pt strain. The TM and TGI results obtained with Mn17181 were confirmed on another locus targeted with Mn17038 ( Supplementary Fig. 1 and Supplementary Tables 1-3 ). Taken together, these results demonstrate the first targeted gene modifications in diatoms. This breakthrough opens new doors for biotechnological applications, notably as regards the re-engineering of diatoms’ lipid metabolism for biofuel production. 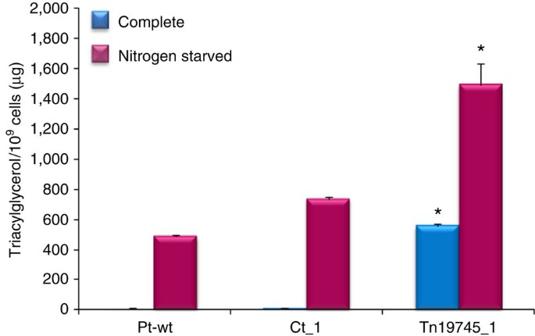Figure 4: Quantification of triacylglycerol content by HPLC-MS/MS. Quantification of TAG content in the Tn19745_1 strain and controls, namely a clone transformed with the plasmid conferring nourseothricin resistance (Ct_1) and the Pt parental strain (Pt wt). The TAG accumulation was assessed in complete versus nitrogen-depleted media. For each sample, a triplicate analysis was performed. For each experiment Tn19745_1 was compared with Pt wt (t-test, *P<0.05) and Ct_1 (t-test, *P<0.05). Data are shown as the mean+s.d. Targeted genome modifications induced by TALEN We then designed TALEN to target genes potentially affecting (i) lipid content (UDP-glucose pyrophosphorylase, Tn19745; glycerol-3-phosphate dehydrogenase, Tn23159; enoyl-ACP reductase, Tn23157), (ii) acyl chain length (long chain acyl-CoA elongase, Tn19746; putative palmitoyl-protein thioesterase, Tn19744) or (iii) the degree of fatty acid saturation (omega-3 fatty acid desaturase, Tn23158; delta 12-fatty acid desaturase, Tn19743) ( Supplementary Table 4 ). TALEN were synthesized using our proprietary TALE array synthesis method described in Supplementary Fig. 2 and Supplementary Table 5 . After assembly, TALEN were tested for their ability to induce TM [30] . Because of low transformation efficiencies in diatoms, we obtained 7 to 62 NAT-resistant colonies per TALEN transformation. For each experiment, the analysis of a subset of colonies (69.1%±20%) revealed that 7 to 56% had gene modification events ( Supplementary Table 6 ). The identification of these events was carried out by PCR amplification surrounding the nuclease target site. Interestingly, several of the colonies obtained after transformation with TALEN Tn23158, Tn19746 and Tn19745 displayed high frequencies (50 or 100%) of large insertions that were directly detectable by electrophoresis of the PCR products on agarose gel. Examples of these events are shown in Fig. 2b . Sanger sequencing of the inserts revealed that they corresponded to fragments of the plasmids used during the transformation ( Supplementary Fig. 3 ). In the absence of noticeable insertions or deletions, the PCR amplicons were subjected to a T7 endonuclease assay [31] ( Supplementary Fig. 4 ). For PCR products cleaved with this assay, the quantification and characterization of the mutagenic events were then performed by deep sequencing. The TM frequencies ranged from 6 to 100% ( Fig. 2a ), and, as shown in Supplementary Fig. 5 , the majority of mutagenic events were deletions or insertions (fewer than 40 bp). Figure 2: Targeted mutagenesis induced by TALE nucleases. ( a ) TM frequency induced by TALEN-targeting genes involved in lipid metabolism and measured by deep sequencing. All the colonies with targeted mutations after transformation with their respective TALEN ( Supplementary Table 4 ) are represented in this graph. Mutations were detected via amplicon sequencing using primers flanking the nuclease target site. For each locus, the control corresponds to a colony transformed with a plasmid carrying the antibiotic resistance gene alone (Ct_1 to Ct_7). ( b ) Examples of mutagenic events induced by TALEN Tn19745, Tn23158 and Tn19746, and directly evidenced by the presence of higher PCR products when compared with their respective controls (Ct_1 to Ct_3). Full size image Generation of an enhanced lipid-producing strain To further study the impact of gene modification on lipid metabolism, we selected the Tn19745_1 strain (UDP-glucose pyrophosphorylase: UGPase) for three main reasons: (i) we were expecting that the inactivation of a gene involved in the carbohydrate storage pathway such as UDP-glucose pyrophosphorylase ( Fig. 3a ) would lead to an increase in triacylglycerol (TAG) accumulation, as previously observed in Chlamydomonas reinhardtii strains with mutations in the ADP-glucose pyrophosphorylase ( AGPase ) gene [32] ; in Phaeodactylum tricornutum , UGPase led to the storage of polysaccharides in chrysolaminarin form; (ii) the lack of wild-type sequences in our PCR screening indicated a complete disruption of the coding sequence, which allowed us further characterization without a subcloning step; (iii) the insertion led to the emergence of a stop codon ( Supplementary Fig. 3 ). Figure 3: Analysis of neutral lipid profiles by flow cytometry. ( a ) Simplified overview of the pathways involved in fatty acid synthesis and chrysolaminarin accumulation. ( b ) Flow cytometry analysis of neutral lipid content in the UGPase knock-out clone (Tn19745_1), a clone transformed with the plasmid for nourseothricin resistance (Ct_1) and the Pt parental strain (Pt wt). This BODIPY profile corresponds to one of the four experiments quantified in c . The graph represents the number of cells as a function of the fluorescence intensity of BODIPY labelling. Vertical lanes delimit, on the left, the fraction of the unlabelled cells, and, on the right, the fraction of cells exhibiting low versus high fluorescence intensity, which refers to cells with low versus high neutral lipid content. ( c ) Quantification of the number of cells with high-lipid content was performed in four independent experiments with Tn19745_1 compared with Pt wt ( t -test, * P <0.05) and Ct_1 ( t -test, * P <0.05). Data are shown as the mean+s.d. Full size image To assess neutral lipid content, we first performed flow cytometry using the specific lipid droplet stain BODIPY 493/503 (ref. 33) [33] ( Fig. 3b ). Analysis of the mutant strain Tn19745_1 showed a strong and reproducible shift in the mean fluorescence when compared with controls, indicating an increase in the ratio of cells with high-lipid content within the population ( Fig. 3b,c ). To confirm this result and quantify TAGs in the Tn19745_1 mutant, we performed a HPLC-MS/MS lipidomic study. Indeed, this clone had 45 times more TAG than controls ( P <0.05) ( Fig. 4 ). This strain is of particular interest to the industry, since the amount of TAG observed was close to that obtained by nitrogen deprivation, a stress commonly used to accumulate neutral lipids [17] . A further increase was observed in TAG production when the Tn19745_1 mutant was grown in nitrogen-depleted medium (three times higher than the Pt wild type, P <0.05) ( Fig. 4 ). Figure 4: Quantification of triacylglycerol content by HPLC-MS/MS. Quantification of TAG content in the Tn19745_1 strain and controls, namely a clone transformed with the plasmid conferring nourseothricin resistance (Ct_1) and the Pt parental strain (Pt wt). The TAG accumulation was assessed in complete versus nitrogen-depleted media. For each sample, a triplicate analysis was performed. For each experiment Tn19745_1 was compared with Pt wt ( t -test, * P <0.05) and Ct_1 ( t -test, * P <0.05). Data are shown as the mean+s.d. Full size image In this study, we developed a highly efficient method for editing the Phaeodactylum tricornutum genome using sequence-specific nucleases. To our knowledge, only one study has reported the modification of the genome of a unicellular green alga; in that study, zinc-finger nucleases were used to modify an artificial reporter gene stably integrated into the Chlamydomonas reinhardtii genome [23] . Here, by targeting seven genes involved in the lipid metabolism of Phaeodactylum tricornutum , we demonstrated high frequencies of TALEN-mediated genome modification in this species, with 7 to 56% of colonies exhibiting TM. Furthermore, we generated an enhanced lipid-producing strain with a 45-fold increase in TAG content when compared with the parental Pt strain cultured in the same conditions. This lipid-producing strain promises to be useful for biofuel production, and the ability to manipulate metabolic pathways using sequence-specific nucleases, in general, will pave the way for synthetic biology in diatoms. Our methods can also be used to further understand the biology of these fascinating microalgae. Diatoms are model organisms for understanding carbon fixation [34] , [35] , light harvesting [36] and lipid [37] and silicon metabolism [38] . The tools of genome engineering can be used to advance diatom biology by allowing for reverse genetics, including gene inactivation, replacement and tagging. Culture conditions The Phaeodactylum tricornutum Bohlin clone CCMP2561 was grown in filtered Guillard f/2 medium [39] (Sigma G0154) without silica, 40‰ Sigma Sea Salts S9883 at 20 °C. The incubator was equipped with white neon light tubes providing illumination of about 120 μmol photons m −2 s −1 and a photoperiod of 12 h light:12 h dark. Liquid cultures were done in vented cap flasks. Engineered nucleases The Mn17181 and Mn17038 MNs used in this study were derived from I-CreI and were engineered using a 2-step semi-rational strategy allowing the complete redesign of endonuclease specificity [40] . The first step consists in identifying collections of variants with locally altered specificity by randomizing specific residues in the DNA-binding domain of the protein, and the second step is based on a combinatorial approach wherein sets of mutants from different locally engineered variants are assembled to create globally engineered proteins with predictable specificity. Further engineering steps may be needed to improve their activity. MNs were used in a single-chain format [41] , which consists in the fusion of two I-CreI-derived variants (monomer left and right) via a peptidic linker. The TALEN were derived from TALE AvrBs3. TALEN™ is a trademark owned by Cellectis Bioresearch. Throughout this study, we used a TALEN scaffold N-terminal domain (full length) and C-terminal domain (+C40). The reverse synthesis method is described in Supplementary Fig. 2 . This method was used to produce eight TALE arrays (four TALEN); the remaining six TALE arrays (three TALEN) were obtained from Cellectis Bioresearch. All information on nucleases is presented in Supplementary Tables 7 and 8 . TALEN synthesis The first step involves the construction of di- and tri-repeat block collections. Each mono repeat unit (HD:C, NG:T, NI:A, NN:G and NG*:T) was commercially synthesized on an individual basis (Top Gene Technologies) and subcloned in the pAPG10 plasmid (Top Gene Technologies). Each of the inserted sequences was flanked by BbvI and SfaNI type IIs restriction sites. The overhang created by these two enzymes was compatible except for the NG* (last half repeat unit) where SfaNI created a unique non-compatible overhang. In addition, a SfiI site was placed on the outside to allow recloning of every construction in the pAPG10 plasmid. All possible 16 di-, 64 tri-repeat units (excluding the one containing NG*) and 4 di-repeat units including NG* were prepared by consecutive restrictions, ligations (using BbvI and SfaNI) and subcloning in the pAPG10 using SfiI, creating a collection of 84 plasmids, which were PCR amplified to generate di/tri-modules for synthesis assembly. For reverse synthesis, biotinylated di- and tri-blocks were amplified by PCR using the primers TAL-shuttle-F-short-Biotin (5′biotin-CCTCACAGGCCGGACGGGCCGAC-3′)/TAL-shuttle-R-short (5′-CCCGGTACCGCATCTCGAGG-3′). Terminal di-blocks (containing NG*) were amplified by PCR using the primers TAL-shuttle-F-short (5′-CCTCACAGGCCGGACGGGCCGAC-3′)/TAL-shuttle-R-short (5′-CCCGGTACCGCATCTCGAGG-3′). Conditions for PCR amplification were typically 5 ng of plasmid template, 250 μM dNTP mix, 200 nM of each oligonucleotide and 1 μl of Herculase II Fusion DNA Polymerase (Agilent) in a final volume of 50 μl of Herculase buffer 1 × . PCR conditions were 5 min at 95 °C, 30 cycles of 30 s at 95 °C, 30 s at 48 °C and 20 s at 72 °C and a final step of 3 min at 72 °C. PCR products were column-purified using a nucleospin extract II kit (Macherey-Nagel) and recovered in 40 μl H 2 0. Initial biotinylated di- and tri-blocks were digested with SfaNI (FastDigest, Fermentas); terminal di-modules were digested with BbvI (FastDigest Lsp1109I, Fermentas). Digested fragments were column purified and quantified (Nanodrop, Thermo scientific). Two micrograms of purified digested PCR products were typically obtained with this process. The assembly procedure started with two washing steps for the streptavidin-coated magnetic beads (5 μl, Dynabeads MyOne Streptavidin T1, Life Technologies) with 100 μl buffer A (TBS 1X, 0.05% TWEEN20) and was further performed as follows (all steps were performed in 50 μl under shaking, 700 r.p.m. ): (1) parallel individual immobilization of the desired SfaNI-digested tri-blocks (100 ng) and di-blocks (70 ng) in buffer A on the streptavidin-coated magnetic beads, 1 h at room temperature followed by three washing steps with buffer B (TBS 1X, 0.05% TWEEN20, NaCl 1 M) and 2 with buffer A; (2) ligation of BbvI-digested terminal di-block (100 ng) in 1X ligation buffer containing 6U of T4 DNA ligase to the desired immobilized di- or tri-blocks at room temperature. After 30 min, 0.5 mM ATP (Fermentas, final concentration) was added and the reaction was set for an additional 30 min, followed by three washing steps with buffer B and 2 with buffer A; (3) release of the nascent chain from the solid surface by addition of BbvI (0.25 FDU, FastDigest Lsp1109I, Fermentas) in 1X Fast digestion buffer, followed by thermal inactivation (65 °C, 25 min) of the restriction enzyme. The reaction was subsequently cooled down to room temperature; (4) ligation of the nascent chain to the desired immobilized (step 1) di- or tri-blocks by addition of the reaction mixture from step 3 complemented with 1X ligation buffer and 6U of T4 DNA ligase. After 30 min, ATP was added as described in step 2; (5) steps 3 and 4 were repeated sequentially using the desired immobilized di- or tri- blocks; (6) after three washing steps with buffer B and 3 more with buffer A, the synthesized chain was released with either SfiI (New England Biolabs) to allow subcloning in the shuttle plasmid pAPG10, or by sequential SfaNI, wash, BbvI digestions to allow subcloning in plasmids already containing a TALEN scaffold. The product was then transformed in XL1b (Stratagene) according to standard molecular biology procedures; (7) selection of clones containing an insert of the desired size was achieved by colony PCR screening using appropriate primers, M13_Forward (5′-GTAAAACGACGGCCAG-3′)/M13_Reverse (5′-CAGGAAACAGCTATGAC-3′) or TAL-Screen-NForA (5′-GCGGGAGAGTTGAGAGGTCCAC-3′) / TAL-Screen-FRevA (5′-CAGGATACGGTCCTGGGTGCTGTTC-3′) for pAPG10 or TALEN backbone plasmid, respectively. Genetic transformations Cells (5 × 10 7 ) were collected from exponentially growing liquid cultures and spread on 10 cm 1% agar plates containing 20‰ sea salts supplemented with f/2 solution without silica. Two hours later, transformations were carried out using the microparticle bombardment method (Biolistic PDS-1000/He Particle Delivery System (BioRad)) adapted from Apt and collaborators [42] with minor modifications. In brief, M17 tungsten particles (particle diameter of 1.1 μm, BioRad) were coated with DNA using 1.25 M CaCl 2 and 20 mM spermidin. Agar plates with the diatoms to be transformed were positioned at 7.5 cm from the stopping screen within the bombardment chamber. A burst pressure of 1,550 psi and a vacuum of 25 Hg were used. For the TM experiments, 1.5 μg or 3 μg of each plasmid encoding the monomers of the TALE nucleases and 3 μg of the NAT selection plasmid were used. The DNA amount was brought to 9 μg using an empty vector plasmid. For the meganuclease experiments, the DNA mixture contained 3 μg of the meganuclease expression vector, 3 μg of the scTrex2-encoding plasmid and 3 μg of the NAT selection plasmid. For the TGI experiments, a total of 9 μg of DNA was used, containing 3 μg of the meganuclease expression vector, 3 μg of the donor matrix and 3 μg of the NAT selection plasmid. The donor matrix was composed of two homology arms of 750 bp each separated by 29 bp of an exogenous sequence, allowing for the detection of mutagenic events and the quantification of the TGI frequency by deep sequencing. The sequence of these 29 bp is described in Supplementary Table 9 . The donor matrix as well as plasmids coding for NAT resistance, scTrex2, the TALEN and the MN were all delivered as circular plasmids. As negative controls, beads were coated with a DNA mixture composed of 3 μg of the NAT selection plasmid and 6 or 3 μg of the empty vector for TM or TGI experiments, respectively. Five bombardments were performed using the mixture of DNA. Two days post-transformation, bombarded cells were spread on 300 μg ml −1 NAT (Werner Bioagents) agar plates and placed in the incubator under a 12 h light:12 h dark cycle for at least 3 weeks. After 3 weeks, colonies were re-streaked on fresh 10 cm 1% agar plates containing 300 μg ml −1 NAT. For subcloning, colonies from transformations were re-suspended in culture medium and plated at a low density (600 cells on a 10 cm agar plate containing NAT antibiotic), enabling the isolation of subclones 2 weeks later. Genotypic characterization Cell lysates from resistant colonies were prepared by dissociation of colonies in 20 μl of lysis buffer (1% TritonX-100, 20 mM Tris–HCl pH 8, 2 mM EDTA) in an Eppendorf tube. Tubes were vortexed for at least 30 s and then kept on ice for 15 min. After heating for 10 min at 85 °C, tubes were cooled down at RT. After a 1:5 dilution in water and a brief centrifugation to pellet cell debris, supernatants were used immediately or stocked at 4 °C. Five microlitres of cell lysates were used for the PCR amplification of the genomic targets with specific primers compatible with NGS sequencing (454 Life Sciences). Sequences of the primers used are presented in Supplementary Table 9 . The PCR products were first analysed by electrophoresis migration on agarose gel. In the event of migration shifts due to insertions, the PCR amplicons were sequenced using the Sanger method (Eurofins MWG Operon). In the absence of noticeable modifications of the amplicon size compared with controls, the PCR products were purified on magnetic beads (Agencourt AMPure XP, Beckman Coulter) and then subjected to T7 endonuclease assay. In brief, 50 ng of the amplicons was denatured and then annealed in 10 μl of annealing buffer (10 mM Tris–HCl pH8, 100 mM NaCl, 1 mM EDTA) using an Eppendorf Master Cycle gradient PCR machine. The annealing program is as follows: 95 °C for 10 min; fast cooling to 85 °C at 3 °C s −1 ; and slow cooling to 25 °C at 0.3 °C s −1 . The totality of the annealed DNA was digested for 15 min at 37 °C with 0.5 μl of the T7 Endonuclease I (10 U μl −1 ) (M0302 Biolabs) in a final volume of 20 μl (1 × NEB buffer 2, Biolabs). Ten microlitres of the digestion was then loaded on a 10% polyacrylamide MiniProtean TBE precast gel (BioRad). After migration the gel was stained with SYBRgreen and scanned on a Gel Doc XR+ apparatus (BioRad). To quantify the frequency of the mutagenic events first evidenced by the T7 endonuclease assay, the same purified PCR products were sequenced using NGS technology (454 Life Sciences). In all, 500–20,000 reads per sample were analysed. The processing of NGS (454 Roche) data was done according to the following procedure: we filtered out sequences that (i) were too short and did not cover the target locus (sequences must have at least 20 bp after the end of the target locus), (ii) had too many off-target site indels (more than 20% of the total sequence length) or (iii) had indels that were likely to be 454 sequencing errors. For this purpose, we built a statistical model that detected sequencing errors based on the following indel features: short indel size (1 bp, indels are likely to be sequencing errors), mononucleic stretches and sequence quality around the indel region. An example of filtering is presented in Supplementary Fig. 6 . For TGI experiments, the detection of targeted integration was performed via specific PCR amplification using one primer located within the heterologous insert of the DNA repair matrix and another located on the genomic sequence outside the matrix homology arms (Screen left and Screen right). The quantification of TGI was performed by deep sequencing. For that, two successive PCR reactions were carried out: the first one (locus specific) was performed using primers outside of the homology arms. The amplification product was then purified on gel, and an aliquot (1/60 of the elution) was used for nested PCR using primers flanked by specific adaptors required for NGS sequencing. BODIPY labelling Cells were re-suspended at a density of 5 × 10 5 cells ml −1 . Labelling was performed at a final concentration of 10 μM BODIPY 493/503 (D-3922 Molecular Probes) in the presence of 10% DMSO for 10 min at room temperature in the dark. Fluorescence intensity was measured by flow cytometry (excitation wavelength 488 nm, emission maximum 515 nm) [33] . Measuring TAG content The lipidomic study was performed by APLIPID ( www.aplipid.com ). Cells were seeded at a density of 2 × 10 5 cells ml −1 in 300 ml of filtered sea water enriched with complete or nitrate-depleted f/2 medium [39] . Three days later, cells were counted with Kova slides (Hycor) and collected on tared filter paper circles. After drying, filters were weighed and lipids extracted according to Bligh and Dyer [43] . The level of molecular species comprised in TAG was assayed by HPLC-MS/MS using a method adapted from Donot and collaborators [44] . TAGs (retention time 9 min) were separated from other neutral lipids and phospholipids (retention time >15 min) on a polyvinyl alcohol functionalized silica column (PVA-Sil, YMC Europe GmbH, Schöttmannshof 19 D-46539 Dinslaken, Germany). Molecular species were monitored by the neutral loss of fatty acid after collision-induced dissociation. For each sample, a triplicate analysis was performed. Statistical analysis A standard Student’s t -test (P-values) was done to compare the number of cells with high-lipid content ( Fig. 3 ) and the TAG content ( Fig. 4 ) between Tn19745_1 strain and its controls Pt wt or Ct_1. How to cite this article: Daboussi, F. et al. Genome engineering empowers the diatom Phaeodactylum tricornutum for biotechnology. Nat. Commun. 5:3831 doi: 10.1038/ncomms4831 (2014).